Optical control of hard X-ray polarization by electron injection in a laser wakefield accelerator Laser-plasma particle accelerators could provide more compact sources of high-energy radiation than conventional accelerators. Moreover, because they deliver radiation in femtosecond pulses, they could improve the time resolution of X-ray absorption techniques. Here we show that we can measure and control the polarization of ultra-short, broad-band keV photon pulses emitted from a laser-plasma-based betatron source. The electron trajectories and hence the polarization of the emitted X-rays are experimentally controlled by the pulse-front tilt of the driving laser pulses. Particle-in-cell simulations show that an asymmetric plasma wave can be driven by a tilted pulse front and a non-symmetric intensity distribution of the focal spot. Both lead to a notable off-axis electron injection followed by collective electron–betatron oscillations. We expect that our method for an all-optical steering is not only useful for plasma-based X-ray sources but also has significance for future laser-based particle accelerators. Laser-plasma-based electron acceleration is the first step towards the generation of spatially and temporally coherent hard X-ray pulses in the femtosecond time domain. Broad-band femtosecond X-ray pulses provide new opportunities for time-resolved X-ray absorption spectroscopy, shedding light on chemical reaction dynamics [1] , [2] or revealing ultra-fast structural changes [3] . The availability of a source with polarized X-rays could pave the way for studying the dynamics of magnetization via linear magnetic dichroism [4] or for studying structural changes in thin films by employing polarization-dependent X-ray absorption fine structure spectroscopy [5] . Polarized X-rays are also widely used in materials science and biology to significantly enhance the sensitivity of X-ray fluorescence analysis [6] . One possible route for generating X-rays is to induce a wiggling motion of the accelerated electrons in a conventional undulator consisting of a periodic magnetic structure like that found in a synchrotron. Using this approach, spatially coherent soft X-rays up to an energy of 200 eV have been generated [7] , [8] , holding the promise for a table-top X-ray-free electron laser [9] . Much more straightforward is applying the strong localized electric and magnetic fields inside the plasma and using the plasma itself as an effective wiggler structure to produce hard X-ray radiation [10] , [11] , [12] . The major advantage of the latter approach is that plasmas can produce multimega-gauss fields [13] and have a much shorter effective wiggler period on the order of a few hundred micrometres [14] , resulting in a low divergence beam of keV X-rays even for electrons in the 100-MeV range. A laser-plasma accelerator can be realized by focusing a femtosecond laser pulse to intensities of ~ 10 19 W cm − 2 into a millimetre-scale supersonic gas jet. When using helium or hydrogen as the target gas the leading edge of the pulse is already intense enough to fully ionize the gas. In the central part of the laser pulse the intensity, and hence the pondermotive potential, is strong enough to push the electrons away from the optical axis and a plasma wave is excited in its wake. This plasma wave, travelling close to the speed of light, can break after strong excitation. As a consequence of this wave breaking, electrons are injected into the plasma-wave structure. The electric field inside the wave is strong enough (≈100 GV m −1 ) to accelerate the electrons in the forward direction to relativistic energies in excess of 1 GeV over distances of only a few millimetres or centimetres [15] . Also present in the plasma wave together with an azimuthal magnetic field is a transverse electric field associated with the charge separation in the plasma wave, forcing the highly relativistic electrons into a transverse oscillation leading to the emission of betatron radiation in the X-ray regime [12] . It was shown that for electrons in an energy range of about 100 MeV the largest number of keV photons is emitted from the region in the plasma where the electrons have the maximum energy [16] . The radiation from the relativistically moving charges emitted into a spectral band dω, centred on the frequency ω, and into the solid angle dΩ centred on the observation direction , is a function of the electron velocity (normalized to the speed of light in vacuum) and the electron trajectory ( t ), and reads [17] where e is the electron charge and ε 0 the vacuum permittivity. Inspecting equation (1) immediately reveals that the polarization state of the output depends on the direction of the electrons’ oscillation in the plane perpendicular to the laser’s propagation direction. In this article, we report on a mechanism to control the off-axis injection of the electrons into the plasma wave, and hence adjust the electron trajectory. One all-optical method is to tilt the pulse front of the driving laser pulse to create a non-symmetric spatio-temporal distribution of the focal spot. For a tilted pulse front the maximum intensity will be reached at different times across the beam profile, breaking the symmetry and preferentially injecting the electrons into the plane of the laser’s tilted pulse front with a spatial offset to the plasma wave’s axis as shown recently [18] . Likewise, an asymmetric laser intensity profile leads to a non-symmetric intensity distribution within the focal plane [19] . Since the laser intensity profile is asymmetric, the radial ponderomotive force is different in each direction, driving an asymmetric plasma wave resulting in a substantial off-axis injection of the electrons [20] . To fully model our experiment we analyse also the emitted X-ray radiation’s polarization state predicted by our three-dimensional particle-in-cell (PIC) VLPL-Code [21] either for different pulse-front tilts or for an asymmetric intensity distribution in the focal spot (see Methods). Numerical results We first carried out PIC simulations for a tilted pulse front and a non-symmetric intensity distribution of the focal spot. Both deviations from a perfect Gaussian beam are expected to inject electrons off-axis into the plasma wave ( Fig. 1 ). As shown by the simulations, without any aberration of the laser beam the injected electrons oscillate about the laser axis with the betatron frequency ( Fig. 1a ) and emit X-ray radiation with no well-defined polarization state. With an additional pulse-front tilt, the electrons are injected off-axis, leading to a larger initial amplitude of the betatron oscillation and a significantly higher number of X-ray photons polarized in the plane of the electrons’ oscillation ( Fig. 1b ). Similar results can be achieved by introducing an asymmetric focal spot ( Fig. 1c ). In summary, the simulations reveal that controlling the off-axis injection of the electrons by tilting the pulse front of the driving laser pulse is a promising method to control the polarization of the X-ray pulses. 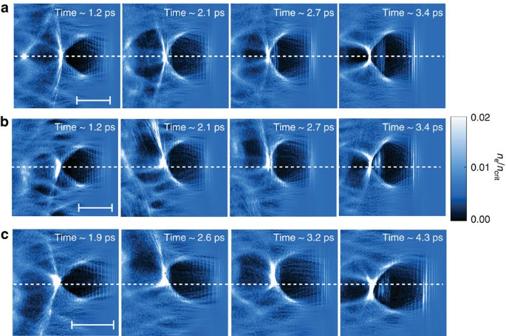Figure 1: Snapshots of the simulated electron density distribution. (a) On-axis electron injection driven by a laser pulse with no pulse-front tilt and an ideal symmetric focal spot. The white scale bar in each figure corresponds to a length of 10 μm. (b) A significant pulse-front tilt showing an asymmetric off-axis injection of the electrons. The dashed line indicates the on-axis position. (c) An asymmetric plasma wave is also driven by a non-symmetric intensity distribution of the focal spot leading to a notable off-axis electron injection and also to collective electron–betatron oscillations. Parameters used in the simulation:ne=1 × 1019cm−3,λ=800 nm, laser spot-diameter 12 μm, laser pulse duration 30 fs and initiallya0=2.0 (experimental case). Figure 1: Snapshots of the simulated electron density distribution. ( a ) On-axis electron injection driven by a laser pulse with no pulse-front tilt and an ideal symmetric focal spot. The white scale bar in each figure corresponds to a length of 10 μm. ( b ) A significant pulse-front tilt showing an asymmetric off-axis injection of the electrons. The dashed line indicates the on-axis position. ( c ) An asymmetric plasma wave is also driven by a non-symmetric intensity distribution of the focal spot leading to a notable off-axis electron injection and also to collective electron–betatron oscillations. Parameters used in the simulation: n e =1 × 10 19 cm −3 , λ =800 nm, laser spot-diameter 12 μm, laser pulse duration 30 fs and initially a 0 =2.0 (experimental case). Full size image Experimental results Experimentally, the pulse front can be tilted by slightly misaligning one of the compressor’s gratings, which are used in a chirped pulse amplification (CPA) laser system [22] . The misaligned grating causes an angular chirp in the spectral domain corresponding to a tilted pulse front in the time domain [23] , [24] . Introducing a pulse-front tilt in this way also changes the direction of the compressed beam, which must be compensated by re-aligning the end mirror in the compressor. In our experiment, the relativistic laser pulse (see Methods) is focused into the leading edge of a pulsed gas jet to generate electron bunches that are able to produce intense X-ray beams due to betatron motion ( Fig. 2a ). The far-field distribution of the accelerated electron bunches was analysed with an aiming screen suggesting a collimated electron beam with a divergence of about 4 mrad in both transverse directions. To characterize the electron and X-ray beams simultaneously, we have removed the aiming screen and analysed the electron energy distribution with a magnetic dipole spectrometer placed farther downstream in the beam path. The single-shot, far-field distribution of the generated X-ray beam was measured with detector 3 (see Fig. 2a ) and showed a Gaussian-like spatial distribution with a divergence of 20±5 mrad (see Supplementary Fig. S1 ). By averaging over 100 consecutive shots we obtained a root-mean-square (r.m.s.) fluctuation of the X-ray beam pointing better than ±3 mrad in the horizontal and vertical directions ( Supplementary Fig. S1 ). Taking into account the efficiency of our X-ray detector we have estimated the number of emitted photons with an energy over 3 keV to be about 5 × 10 7 X-ray photons per shot. In the literature, polarization of the X-ray beam has been predicted by analysing the far-field distribution of the electrons [25] ( Supplementary Fig. S2 ) or X-rays [26] , [27] . However, in our experiments the sub-30 fs laser pulses were slightly shorter than the excited plasma wavelength and will be further shortened by an additional longitudinal pulse compression mechanism [28] . According to the theory we can then exclude an interaction of the accelerated electrons with the trailing edge of the laser pulses ( Supplementary Discussion ). To analyse the polarization of the betatron emission we used a single-shot polarimeter ( Fig. 2b ). The polarizer is based on two mutually perpendicular, plain lithium-fluoride (LiF) mosaic crystals. Polarization-sensitive reflection is realized by fulfilling the Bragg condition at Brewster’s angle ( α B ), which is close to 45° for a refractive index of n ≈1 for radiation in the X-ray spectral range (see Methods) [29] . Taking into account the lattice distance of the LiF crystals, only σ -polarized X-ray radiation at 4.35 keV will be reflected and detected with an X-ray-sensitive CCD camera. The extinction ratio of the polarization state measurement between the π -component and the σ -component was calculated to be better than 1:33. The two crystals are sufficiently far away from the X-ray source (4 m) and sufficiently close to each other, ensuring a uniform illumination of both crystals. 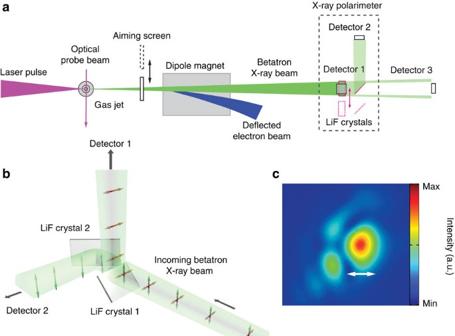Figure 2: Setup of the single-shot X-ray radiation’s polarization state analyser. (a) Anf/13 off-axis parabolic mirror focuses the laser pulses (730 mJ, 27 fs, 800 nm) to a 12-μm-diameter spot into a hydrogen gas jet with 2.7 mm opening diameter. The laser-accelerated electrons were analysed with an aiming screen and a magnetic dipole spectrometer. The betatron X-ray beam was measured with different CCD detectors (labelled as detector 1, 2 and 3). (b) Setup of the single-shot X-ray polarimeter. Two lithium-fluoride crystals are oriented at Brewster’s angle, reflecting either the horizontally (crystal 1) or vertically (crystal 2) polarized X-ray component at 4.35 keV. The two orthogonal polarization components are detected simultaneously with two X-ray CCD cameras (labelled as detector 1 and 2). (c) Having an asymmetric laser focal spot without a deformable mirror generates an asymmetric wakefield. The white double arrow indicates a width of 12 μm. Figure 2: Setup of the single-shot X-ray radiation’s polarization state analyser. ( a ) An f /13 off-axis parabolic mirror focuses the laser pulses (730 mJ, 27 fs, 800 nm) to a 12-μm-diameter spot into a hydrogen gas jet with 2.7 mm opening diameter. The laser-accelerated electrons were analysed with an aiming screen and a magnetic dipole spectrometer. The betatron X-ray beam was measured with different CCD detectors (labelled as detector 1, 2 and 3). ( b ) Setup of the single-shot X-ray polarimeter. Two lithium-fluoride crystals are oriented at Brewster’s angle, reflecting either the horizontally (crystal 1) or vertically (crystal 2) polarized X-ray component at 4.35 keV. The two orthogonal polarization components are detected simultaneously with two X-ray CCD cameras (labelled as detector 1 and 2). ( c ) Having an asymmetric laser focal spot without a deformable mirror generates an asymmetric wakefield. The white double arrow indicates a width of 12 μm. Full size image With this arrangement we are able to simultaneously measure the amount of horizontally and vertically polarized X-ray radiation for each laser shot. Having the possibility to measure the polarization state in a single shot is important to be insensitive to shot-to-shot fluctuations. This is particularly important as the output signal depends critically on the exact position of the nonlinear wave breaking, that is, the electron injection position and the inevitable intensity fluctuations within the asymmetric laser focus ( Fig. 2c ). However, with our experimental setup we are not only able to measure the polarization state for each laser shot, but we managed to record for each shot a shadowgraphic image of the plasma wave, the electron spectrum, and the transverse electron beam profile in one dimension. These simultaneously recorded data sets allowed correlation of the polarization states to the electrons’ energy spectra. Here we take advantage of the fact that our electron spectrometer disperses the electron pulse along the horizontal axis, whereas the signal is spatially resolved in the vertical direction [20] . This feature can be used to determine the direction of the off-axis injection of electrons into the plasma wave by tilting the pulse front of the laser pulse [18] . As the X-ray photons are mainly emitted from high-energy electrons [16] , it is sufficient to show the electron spectra only above 60 MeV ( Fig. 3 ). Some shots show a corrugated trace of the electrons on the scintillating screen ( Fig. 3a–c ), while others exhibit a narrow transverse distribution ( Fig. 3d–f ). Many results of the laser–plasma interaction will vary from shot to shot depending on the exact longitudinal and transverse injection position of the electrons. These include the net acceleration length of the electrons, their energy, the plane of the betatron oscillation and the X-ray radiation’s polarization state. The main contributing effect for our setup is the self-injection of electrons due to an asymmetric intensity distribution inside the focal spot, which is likely to vary from shot to shot as well ( Fig. 2c ). Furthermore, we can conclude that in our acceleration regime the betatron polarization state is independent of the direction of the laser’s polarization state, which was not changed during the experiment. The laterally smooth electron distribution can be explained by electrons oscillating mainly in the horizontal direction, while the corrugated structure indicates an additional collective wiggling of the electrons in the vertical direction. For the wiggled electron trace the X-ray signal is primarily vertically polarized ( Fig. 3a–c ), whereas for the straight electron trace we detect mainly horizontally polarized X-rays ( Fig. 3d–f ). As the polarization of the emitted betatron radiation is determined by the plane of oscillation of the electrons injected into the plasma wave, the measured X-ray polarization provides us additional information about the injection of the electrons into the plasma wave. 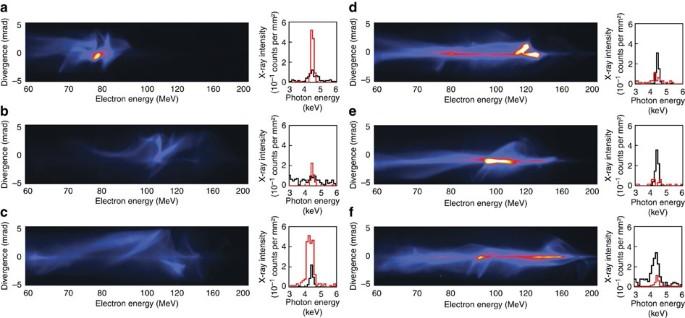Figure 3: Electron spectra and simultaneously measured X-ray polarization state. Typical single-shot electron spectra on the high-energy scintillating screen exhibit (a–c) either a corrugated trace (d–f) or are vertically well confined. For the wiggled electron traces (a–c), the X-ray radiation is mainly vertically polarized (red line) and have only a minor contribution in the horizontal polarization direction (black line). For the vertically confined electron traces (d–f) the horizontally polarized component dominates. The photon number within only one Bragg peak corresponds to nearly 103photons per shot. The shot-to-shot fluctuations are attributed to the asymmetric intensity distribution inside the focal spot, which varies from shot to shot as well. Figure 3: Electron spectra and simultaneously measured X-ray polarization state. Typical single-shot electron spectra on the high-energy scintillating screen exhibit ( a – c ) either a corrugated trace ( d – f ) or are vertically well confined. For the wiggled electron traces ( a – c ), the X-ray radiation is mainly vertically polarized (red line) and have only a minor contribution in the horizontal polarization direction (black line). For the vertically confined electron traces ( d – f ) the horizontally polarized component dominates. The photon number within only one Bragg peak corresponds to nearly 10 3 photons per shot. The shot-to-shot fluctuations are attributed to the asymmetric intensity distribution inside the focal spot, which varies from shot to shot as well. Full size image To overcome the shot-to-shot fluctuations of the polarization state of the betatron emission it is necessary to control the off-axis injection of the electrons into the plasma wave. Therefore we increased the spatio temporal asymmetry within the focal spot by introducing a vertical pulse-front tilt, which was sufficient to overcome the statistical fluctuations. In Fig. 4a we present an image of the plasma wave taken with the probe beam that crosses the plasma at an early stage in the interaction. The gas jet is placed in front of the focal position of the main laser pulse propagating from the left to the right. The intensity modulation (grey scale) can be associated with the plasma wave and exhibits a very strong tilt against its propagation direction. It is important to mention that the shadowgram does not directly show the electrons’ density distribution. The observed spatial intensity modulation is created from the spatially homogeneous probe pulse refracting through the electrons’ density modulation inside the plasma. Light and dark areas in the image are formed proportional to the Laplacian of the plasma’s refractive index [30] . From this image we can estimate a wavelength of the plasma wave on the order of 15 μm, corresponding to an electron density of 5 × 10 18 cm −3 . This is in good agreement with the calculated density derived from interferometric characterization of the nozzle using a neutral gas [31] . The effect of this introduced pulse asymmetry on the polarization of the betatron emission is depicted in Fig. 4 averaged over 100 consecutive laser shots. 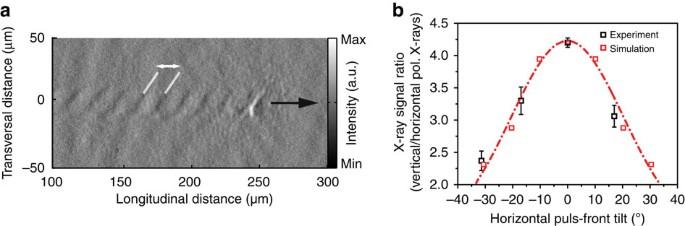Figure 4: Controlling the X-ray polarization by tilting the pulse front. (a) Snapshot of the electron density gradient taken with a 6-fs duration probe pulse for zero horizontal angular dispersion. The laser pulse propagates from left to right and the plasma wave is vertically tilted due to a spatio-temporal asymmetry of the focal spot. We increase oura prioriasymmetric intensity distribution within the focus to rule out shot-to-shot fluctuation of the X-ray polarization state, which was sufficient to overcome the statistical fluctuations. The white double arrow indicates a length of 15 μm. (b) Ratio of the vertically and horizontally polarized X-ray contribution as a function of the horizontal angular dispersion of the laser pulse. Each data point corresponds to an average over at least 100 consecutive shots, and the error bars indicate the standard error of the mean value (black squares). Our measurements fit very well to the predictions from the 3D PIC simulations (red squares). The red dashed line is to guide the eye. Figure 4: Controlling the X-ray polarization by tilting the pulse front. ( a ) Snapshot of the electron density gradient taken with a 6-fs duration probe pulse for zero horizontal angular dispersion. The laser pulse propagates from left to right and the plasma wave is vertically tilted due to a spatio-temporal asymmetry of the focal spot. We increase our a priori asymmetric intensity distribution within the focus to rule out shot-to-shot fluctuation of the X-ray polarization state, which was sufficient to overcome the statistical fluctuations. The white double arrow indicates a length of 15 μm. ( b ) Ratio of the vertically and horizontally polarized X-ray contribution as a function of the horizontal angular dispersion of the laser pulse. Each data point corresponds to an average over at least 100 consecutive shots, and the error bars indicate the standard error of the mean value (black squares). Our measurements fit very well to the predictions from the 3D PIC simulations (red squares). The red dashed line is to guide the eye. Full size image To reduce the effect of fluctuations of the X-ray’s intensity between measurements of different pulse-front tilts we plotted the ratio of the spectrally and temporally integrated signal in the vertical plane to the horizontal plane. The spectral integration spans the high reflectivity range of the LiF crystal in the range of 4.2–4.5 keV. Here, for an asymmetry within the focal spot mainly in the vertical direction, a net ratio of 4:1 for vertical polarized X-rays arises. The vertically tilted pulse front, which mainly causes self-injection of electrons with a vertical offset, resulted in vertically polarized X-rays. To demonstrate the influence of the tilt, we rotate one of the compressor gratings in the dispersive plane away from the position without angular tilt, which results in a horizontal angular dispersion. This favours injection in the plane with the tilted pulse front (horizontal plane) and this ratio starts to decline, in agreement with our theory. However, it is not possible to completely invert the intensity ratio because the electron acceleration becomes more and more inefficient due to the longer pulse duration of the laser pulse within the focal spot. Fig. 4b reveals the strong impact of the tilt on the polarization state. With increasing horizontal tilt, the electrons are injected with a higher probability off-axis in the horizontal direction, which increases the number of horizontally polarized X-rays. This measurement demonstrates the feasibility to control the X-ray’s polarization with an all-optical method, and is in excellent agreement with our predictions based on 3D PIC simulations. By controlling the injection of the electrons in a laser wakefield accelerator, we have demonstrated that we can tune the polarization state of the emitted X-rays. The simulation results obtained here indicate that a non-symmetric plasma wave can be driven by tilting the pulse front of the driving laser pulse or by inducing a non-symmetric intensity distribution of the focal spot. Both methods result in a notable off-axis injection of the electrons and also result in the generation of pulsed X-rays polarized either in the plane of the tilted pulse front or in the plane of the focus asymmetry, depending on the method used. Our measurements reveal the importance of controlling the injection of the electrons into the plasma wave with regard to the resulting X-ray polarization state. We also show that we can influence the direction of an additional transverse momentum of the accelerated electrons, which will be of importance for feeding the electrons into an additional conventional accelerator or a permanent magnet-based undulator for generating X-ray radiation. To further increase the polarization purity and sustainable control of the polarization direction, it might be advantageous to work in the harmonically resonant betatron regime, [32] where the electrons’ trajectory can be controlled via the laser polarization itself. Laser-plasma wakefield accelerator The experiments were carried out at the multi-TW, Ti:Sapphire, chirped pulse amplification (CPA) laser system (JETI) in Jena, Germany, delivering 27-fs pulses with an on-target energy of 730 mJ at a central wavelength of 800 nm. The pulses were focused with an f /13 off-axis parabolic mirror into the leading edge of a pulsed supersonic hydrogen-gas jet. The jet consists of a pulsed valve and a conically shaped nozzle with a diameter of 2.7 mm resulting in an adjustable peak electron density of 0.2–2.0 × 10 19 cm −3 , which can be adjusted by varying the backing pressure of the gas. Without a deformable mirror we obtain an asymmetric focal spot of 12 μm diameter at full-width at half-maximum (FWHM), which leads to an intensity of 7.2 × 10 18 W cm − 2 (FWHM) corresponding to a normalized amplitude of the vector potential, a 0 ⩾ 1.9. For most of the experiments the laser was operated in single-shot mode, but operation up to 0.5 Hz was possible, limited only by the read-out time of the X-ray detectors and the gas load in the vacuum chamber. Electron beam diagnostic The laser-accelerated electrons were monitored with scintillating phosphor screens. The first screen, called the aiming screen, was placed after the laser–plasma interaction and analysed the electrons’ single-shot far-field distribution, their pointing and their beam divergence. When the screen was removed, the electrons could enter a magnetic dipole spectrometer (0.7 T over 20 cm), which deflected the electrons depending on their energy onto two different scintillating screens optimized for detecting electrons in the range 10–55 and 60–350 MeV, respectively. The fluorescence of each screen was imaged onto a high-resolution 12-bit Basler A102f CCD camera. X-ray beam diagnostic The X-ray radiation in the laser’s forward direction was detected with two thermoelectrically cooled, back-illuminated, deep-depletion X-ray CCD cameras (ANDOR DO-936NMOW-BR-DD and ANDOR DV420-BR-DD). The residual laser light and the low-energy X-ray radiation (below 1 keV) were blocked by a permanent 50-μm Be-filter placed in front of the DO-936 CCD and a 30-μm Be-filter placed in front of the DV420 CCD. For the polarization measurement we used the CCD cameras in a single-photon counting mode as an energy-sensitive X-ray spectrometer with an energy resolution better than 100 eV. Plasma imaging For the transverse time-resolved optical probing, a fraction of the main laser pulse is further shortened by first broadening the spectrum in a argon filled hollow core fibre and then compressing it with chirped mirrors down to 5.9±0.4 fs. In our experiment the ultra-short pulses at a central wavelength of 750 nm have been used to image the plasma’s density via shadowgraphy, relying on the dependence of the refractive index of the plasma as a function of the electron density. X-ray polarimeter The X-ray polarimeter consists of two LiF crystals using the strongest Bragg reflection 200. For ideal mosaic crystals, the diffracted polarization components with the electric field components parallel ( π -component) and perpendicular ( σ -component) to the diffraction plane are defined by the incident and diffracted wave vector amount cos 2 (2 θ ) and 1, respectively [33] . The 200 netplane distance (2 d 200 =4.027 Å) fits perfectly to the maximum of the betatron spectrum at 4.6 keV by using the Bragg condition ( λ =2 d hkl sin θ , where λ is the reflected wavelength and d hkl the lattice distance of the crystal reflection with hkl being the diffraction indices) close to the Bragg angle of 45°. At this Bragg angle only linearly σ -polarized X-rays are diffracted. The crystals were selected for high crystalline perfection, defined by small angles between the crystal grains. In order to increase the diffraction efficiency, the crystals’ perfection was reduced by a specially controlled grinding procedure. With this treatment the crystals provide integrated reflectivities that are more than nine times higher than for a perfect crystal. The reflectivity over the whole crystal's area was determined to be constant within 6%. The FWHM of the experimentally determined rocking curves yield an energy resolution of 13–22 eV at 4.6 keV photon energy. Both crystals were built into the polarimeter so that their dispersion planes were mutually perpendicular, allowing detection of the vertical and horizontal polarization states of the betatron radiation with an extinction ratio of 1:33 (3.5%). This assumes an alignment accuracy better than 1° for the Bragg angle and uses the measured divergence of the radiation and width of the crystals’ reflection curves. Numerical modelling For predicting the polarization state of the emitted radiation we carried out numerical simulations using the three-dimensional PIC code VLPL [21] . We modelled a linearly polarized laser pulse with a normalized, relativistic amplitude a 0 =2.0, travelling through an underdense plasma of density n =0.01 n cr , with n cr being the critical density for this laser pulse. Our 3D PIC simulations included the recoil force acting on an accelerating electron caused by the emitted radiation (radiation reaction), during which we also derived the polarization state of the emitted radiation by using the changes in the momentum of the emitting particles. We simulated different tilts of the laser’s pulse front and analysed the results for the corresponding values of the electrons’ off-axis injection points ranging from on-axis injection (zero angular dispersion, no pulse-front tilt) to a significant off-axis injection (angular dispersion). How to cite this article: Schnell, M. et al. Optical control of hard X-ray polarization by electron injection in a laser wakefield accelerator. Nat. Commun. 4:2421 doi: 10.1038/ncomms3421 (2013).